Modeling the process of human tumorigenesis Tumorigenesis viewed as an evolutionary process The concept that almost all human tumours represent aberrant clonal outgrowths is well established [3] . However, this simply means that the malignant population that ultimately appears represents the deregulated growth of a single cell. It does not imply biologic or even genetic identity among its progeny. Nevertheless, it does make it likely that all members of the clone will carry a trace of the earliest genetic or epigenetic changes that drove its deregulated expansion. It is also important to remember that, by the time a cancer is first detectable, it will already contain many millions or even billions of cells produced through dozens of amplifying divisions. During this process, additional genetic diversification and evolution occurs ( Fig. 1 ). This is due in part just to normal rates of incorrect DNA replication (estimated as 2.3 × 10 −8 mutations per nucleotide per cell generation in human cells) [4] . A decreased control of DNA stability is also a common feature of malignant cells. Other mechanisms that contribute to the variable diversification of malignant clones include the tissue and genotype of the cell in which the process of transformation is initiated, the age of the individual in which this process begins and numerous environmental factors [5] , [6] , [7] , [8] , [9] . 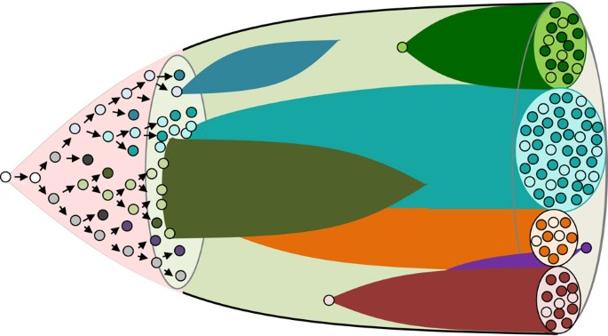Figure 1: Schematic depiction of the subclonal evolution and diversification of cell types in developing malignant populations. In this diagram, subclones identified by accumulating genetic changes are shown by different colours. Cells within each clone that have proliferative potential are shown as pale cells in contrast to some of their progeny that can no longer divide that are shown as dark cells (to illustrate the diversification of biological properties that occurs both within and between subclones), with some clones being transient, whereas others are persistent but variably expanding. Figure 1: Schematic depiction of the subclonal evolution and diversification of cell types in developing malignant populations. In this diagram, subclones identified by accumulating genetic changes are shown by different colours. Cells within each clone that have proliferative potential are shown as pale cells in contrast to some of their progeny that can no longer divide that are shown as dark cells (to illustrate the diversification of biological properties that occurs both within and between subclones), with some clones being transient, whereas others are persistent but variably expanding. Full size image Modern sequencing data has now revealed the enormous heterogeneity that exists within the genomes of malignant populations [10] . This heterogeneity is often apparent within a single cancer assessed at a single moment and sampled from a single site. Additional heterogeneity may also be encountered when different sites are examined, or the same tumour is sampled at different times, or from different individuals with tumours that have arisen in the same tissue. The genetic diversity that characterizes many malignant populations has multiple causes. One is that the full transformation of human cells relies on the accumulation of multiple mutations through a stepwise process in which different rare mutations and/or epigenetic changes must be accrued in order for cells to acquire a deregulated ability for unlimited division as well as other abnormal phenotypic properties [11] , [12] . From this concept, it has been inferred that the process of spontaneous oncogenesis in humans would most often be slow, at least initially, spanning a period of several years. Such a model, in turn, implies that most cancers would originate in a cell type that is normally long-lived but still has sufficient proliferative capacity to accumulate the number of rare mutations required to become transformed. Interestingly, it also implies the possible generation of neoplastic clones with mutations that predispose to further transformation but may never do so, as is being increasingly documented in many tissues [13] , [14] , [15] . However, accelerating the process, and a cause of more rapidly increasing genetic diversity, would be the acquisition of one or more mutations or epigenetic changes that compromise genomic stability [16] , [17] , [18] , [19] . At the same time, recent genomic analyses of some human cancers are suggesting alternative trajectories in which transforming populations early on may undergo cataclysmic bursts of genomic diversification [20] . Most of our knowledge of the process of oncogenesis in human tissues has been derived historically from 3 different types of investigation: (i) genomic analyses of cells obtained from patients at different times during the development and evolution of their cancer with retrospective inferences drawn from the spectrum and prevalence of sequence changes (best determined at the single cell level) [21] , [22] , [23] , [24] ; (ii) inferences derived from single cell or clonal transcriptome studies [25] , [26] ; and (iii) studies of genetically engineered malignant populations in model organisms, and mice in particular [27] , [28] , [29] . The first two of these types of investigation have shown that most human cancers, by the time they become clinically evident, consist of cells that have already acquired multiple mutations [2] . However, the extent to which the time course or order in which the same mutations or other relevant (for example, epigenetically determined) changes are accrued in any given human cancer still remains poorly understood [30] . Although, mutations do not occur randomly [31] , [32] , [33] , the likelihood of a given complement of mutations being accrued in the lifetime of an individual human cell or its progeny remains low. It is therefore not surprising that the more primitive cells in tissues of high cell turnover; that is, those cells responsible for sustaining the required cell outputs of the tissue, have commonly been assumed to serve as reservoirs of premalignant changes that accrue throughout life. In the human hematopoietic system, this concept has been most strongly supported by genomic analyses of cells from patients with chronic myeloid leukemia (CML). This leukemia is unusual in that it is typically diagnosed at an early stage (referred to as chronic phase). Although the clone can already be huge (typically more than a trillion cells), the process of differentiation is minimally perturbed and hence most of the cells are actually highly differentiated, short-lived mature blood cells, indistinguishable from their normal counterparts. Cell production within the chronic phase clone, in fact, largely mirrors the normal process of adult human hematopoiesis and is likewise sustained by a phenotypically similar and rare subset of multi-potent self-renewing CML ( BCR-ABL1+ ) cells as shown by their unique capacity for prolonged CML cell output both in vitro and in vivo [34] , [35] . Interestingly, effective treatment of CML patients with tyrosine kinase inhibitors (TKIs) selectively eliminates the bulk of the clone (>99.9%), but has less effect on the CML stem cells which can then rapidly regenerate an enlarged derivative population if TKI administration is transiently arrested [36] . Moreover, if the chronic phase clone is not adequately reduced, subclones of CML cells with additional mutations and biological properties eventually appear and produce an inevitably fatal acute lymphoid or myeloid leukemia [37] . Additional studies have suggested that at least some other forms of human acute myeloid leukemia (AML) [23] , [38] , [39] , [40] , [41] , [42] myelodysplastic syndromes (MDS) [43] , [44] fit a similar model of step-wise disease progression. The cancer stem cell concept The restriction of transplantable tumour-initiating ability (in immunodeficient mice) to a rare, prospectively separable subset of malignant human cell populations was first demonstrated in human AML [45] . This was followed soon thereafter by analogous experimental evidence of tumour-initiating ability confined to distinct and prospectively separable subsets of cells in primary samples of human breast [46] , brain [47] and colon cancers [48] . Together, these findings established the concept of cancer stem cells thus identified by their transplantable tumour-initiating property. Phenotypic and transcriptional similarities between the subsets of malignant human cells and the stem cells of the tissue of origin have reinforced the association of this ‘cancer stem cell’ functionality with the retention or reactivation of molecular mechanisms essential to the maintenance of normal tissue stem cells. Of particular interest in this regard, has been an association of quiescence with many types of both normal and cancer stem cells [49] , [50] , [51] , [52] , [53] , thus accounting for the innate resistance of the cancer stem cell population to standard chemotherapeutic agents that primarily target dividing cells. The relative insensitivity of these cells to treatment also makes them dangerous reservoirs for the accumulation of additional mutations that make their elimination even more problematic. However, in other human cancers, like melanoma [54] , a majority of the cells with self-sustaining tumorigenic properties is often already apparent at diagnosis. In addition, there is increasing evidence of the reversibility of the properties that confer transplantable tumour-initiating activity in a growing number of human tumours. This phenomenon, referred to as phenotypic instability or plasticity, is thought to reflect changes triggered by cues from the environment or stochastically regulated intrinsic parameters [55] , [56] , [57] , [58] , and may add significantly to the heterogeneous dynamic evolution of tumours caused by a stepwise and branched process of mutation accrual noted already. Transgenic mouse models of de novo tumorigenesis Mouse models have been valuable for analysing early oncogenic events because of the ease with which their genomes can be genetically manipulated in defined manners and times. This has made it possible to interrogate many specific molecular, cellular and tissue-specific characteristics associated with inherited and somatically acquired mutations in humans that have been inferred to play a role in their transformation. There are, however, numerous physiological differences between mice and humans that limit the utility of this approach to provide insights into mechanisms operative in humans. Of particular note in this regard is the apparent ease with which mouse cells can be transformed, in contrast to their human counterparts [59] . Mouse models have been particularly helpful in tracing the clonal origin of normal and transformed cells in various tissues. This type of experiment typically takes advantage of a known lineage-specific gene promoter to transgenically engineer the expression of an oncogene exclusively in the cell types in which that promoter is active. This strategy can thus be used to track subsequent changes in predefined cell types before the formation of a detectable tumour. In addition, this strategy has been useful for identifying the origin of any malignant populations ultimately obtained and demonstrating different properties in the tumours thus generated [27] , [60] , [61] , [62] , [63] . For example, in the adult mammary gland, the specificity of expression of different types of cytokeratins associated with either basal or luminal mammary epithelial cells has enabled tumours derived from these different cell types to be produced and compared. These include the production of estrogen receptor-positive and progesterone receptor-positive (ER + PR + ) and ER − PR − tumours from mouse basal and luminal cells engineered separately to express PIK3CA (H1047R), thereby creating models that appear to mirror analogous phenotypes of human breast cancer [64] , [65] . However, it is also noteworthy that potent stimulation of normal adult mouse luminal mammary cells, even in the absence of a mutant gene, can induce their production of both basal and luminal progeny [66] , despite evidence of their more restricted differentiation behaviour in vitro and in vivo [67] , [68] . Similar transgenic models have been used to study concomitant PIK3CA expression and p53 deletion [64] , [65] , [69] , as well as concomitant BRCA1/PTEN/p53 depletion in mouse mammary cells [70] . Familial adenomatous polyposis, a human condition with a recognized step-wise process of transformation, is another interesting example of a tumour that has been modelled in mice. In this case, the inducible loss of only one APC allele in Lrig1-expressing cells resulted first in their acquisition of pre-neoplastic changes and then their generation of multiple colonic tumours within 50 days [71] . In the epidermis, Sox2 expression has been found to initiate the de novo growth of a squamous cell carcinoma [72] , and glioblastoma in the brain [73] . On the other hand, forced expression of Sox9 in the epidermis was sufficient to induce the de novo formation of basal cell carcinomas [74] . Mouse models have been similarly used to study the ability of Wnt-activation [75] , oncogenic Ras [76] , Myb [77] , and Pgc-1b [78] to initiate de novo tumorigenesis in intestinal epithelial cells. Studies in the hematopoietic system of mice have also reported analogous strategies for the de novo generation of AML [79] , plasma cell neoplasms [80] , and lymphoid malignancies [81] . A key advantage of such transgenic mouse models of oncogenesis is their ability to mimic the effect of acquiring endogenous oncogenic mutations under homeostatic conditions. They also enable events critical to the initiation of tumour formation within the normal tissue architecture to be examined. However, it is also possible that the level of oncogene expression driven by promoters of lineage-specific (tracer) genes would be different from that characteristic of tumours caused by mutations in the corresponding endogenous genes. The different epigenetic mechanisms regulating their expression in the two different sites would be expected to contribute to the types, or at least speed, of the phenotypic changes induced. Furthermore, interactions of spontaneously arising mutant human cells within their native microenvironments, as well as intrinsic aspects of the process of normal tissue control, may not be well modelled in the mouse. On the other hand, transgenic mouse models offer the advantage that they can now be readily engineered to regulate not only the lineage, but also the level, timing and duration of expression of genes of interest that have been introduced into the germ line. Mouse knock-in (KI) protocols now enable some of the short-comings of historic transgenic models to be addressed. These involve the use of homologous recombination to replace endogenous genes in mouse embryonic stem cells with candidate oncogenic mutant alleles and subsequent introduction of the selected cells into the mouse germ line. KI mice have thus been generated to explore the function of Kit mutations in gastrointestinal stromal tumours, the role of TP53 in Li-Fraumeni syndrome tumours and for recapitulating familial cancers. This technique has also been further adapted to induce spontaneous expression of the oncogenic KRAS ( G12D ) gene enabling the genesis of lung cancer, thymic lymphoma, and aberrant intestinal crypt foci to be created and studied [82] . CRISPR/Cas9 technology to introduce oncogenic mutations into the endogenous locus of the mouse germ line (with or without controlled expression) is now offering even greater precision in the types of genetic manipulations that can be deployed to analyse downstream biological effects [83] , [84] , [85] . Transformation of human cell lines Much of the process of malignant transformation of human cells has historically focused on immortalized non-tumorigenic human cell lines as the starting material. MCF-10A is an example of a human mammary epithelial cell line of this type that has been used for this purpose. Forced over-expression of MYC [86] , EGFR [87] , Nicastrin [88] , ERBB2 (ref. 89 ), and RANK [90] in MCF-10A cells produced several phenotypic changes associated with transformation. These included changes in their growth properties in three-dimensional (3D) cultures [91] , as well as in xenotransplant models [89] . However, a study based on a non-tumorigenic human prostate cell line, EPT2-D5, showed that metastatic prostate tumours could be generated in xenografted mice simply by first culturing the cells in a protein-free media to generate ‘spheres’ [92] . Moreover, recent epigenomic and transcriptional analysis of MCF-10A and two other immortalized (184-hTERT) non-tumorigenic human mammary cell lines has revealed that all three have acquired significant differences from primary sources of human mammary cells [93] . It thus remains unclear how well the transformation of such immortalized cell lines will reflect those relevant to the spontaneous genesis of cancers from primary sources of human cells. External factors It is also now clear that most malignant cells are not capable of autonomous growth, although the acquisition of autocrine properties and other intrinsic mechanisms for enhanced auto-stimulation and survival are common. Tumours, like normal tissues, also require a blood supply and frequently contain numerous other non-clonally derived cell types, even to the point where these latter cell types may become predominant [94] , [95] , [96] . These cells may include many different stromal cell types as well as the components of vessel walls and extravasated blood and lymphoid cells. External cues emanating from these different sources both positively and negatively regulate the local rate of growth of neighbouring malignant cells as well as their invasive behaviour [97] , [98] , thereby contributing to the overall dynamic evolution of the genomic, biologic and geographic properties of the entire population of malignant cells [10] . Persistence of tissue-specific programs In addition to these multiple sources of cellular heterogeneity, malignant populations also frequently retain many of the distinguishing but heterogeneous features of the tissue from which they have arisen even after they have metastasized. In fact, almost by definition, a stepwise model of transformation would imply that this would have to be the case unless it completely froze the state of the first affected cell resulting in the generation of a clone of identical daughter phenotypes. If not, then it would be predicted that the composition of a malignant clone would also reflect some of the phenotypic heterogeneity determined by persisting elements of processes that normally sustain the maintenance, organization and differentiation of cells in that tissue [99] . Thus, the phenotypic heterogeneity inherent in many bulk malignant populations would be anticipated to also reflect some of the complex diversity of persisting epigenetic and transcriptional elements characteristic of the formation and maintenance of the tissue from which the cells arose. In this regard, it is noteworthy that different tissues make different utilization of multiple, albeit overlapping basic mechanisms that ultimately co-ordinate their proliferative capacity, survival and epigenetic control of lineage restriction to ultimately establish non-dividing or nonviable cell states. Within the same tissue, these may also change during development and aging as well as under different conditions of homeostasis, wounding, inflammation and infection. Even at a single moment in time, there may be multiple pathways by which a single mature cell type can be generated. Moreover, the properties of ‘self-renewal’ and long-term quiescence in normal cells are now known, at least as suggested by lineage tracing studies in mice, to be more broadly distributed and less rigidly associated with the capacity to regenerate the entire tissue [100] , [101] , [102] . These issues are important because they have necessitated a modification to the historic assumption as to the singular state of ‘stem cells’ even within a given tissue. Hence a greater diversity of cell types can now be envisaged as potential initial cells in which the genetic and epigenetic changes, required to generate irreversibly expanding malignant clones, might originate. As detailed below, these considerations also undermine assumptions underpinning the historic concept of a cancer stem cell, without negating it altogether—a difficult development that the field has now had to accommodate [10] . De novo human models of tumorigenesis Experimental models of de novo tumorigenesis starting from cells isolated directly from normal human tissues are attractive because they circumvent the concerns inherent in extrapolating from immortalized cell line data or species differences ( Fig. 2 ). However, the frequency of success has thus far been much more limited, perhaps due to a historic lag in the development of appropriate methods to isolate the relevant target cells in viable form, and/or to transduce them at an adequate efficiency. Indeed, where these issues have been carefully addressed, some models have been generated ( Table 1 ). For example, normal human basal prostate cells transduced with a combination of vectors encoding cDNAs for AKT , ERG and the androgen receptor have been found to produce tumours in transplanted immunodeficient mice [103] . In contrast, in the same study, transplants of co-isolated luminal prostate cells transduced with the same vectors did not yield tumours. This result is interesting because the gene expression profile of prostate cancers appears closer to that of the luminal cells of the normal prostate. One explanation is that prostate cancers in which these genes are characteristically altered actually originate in basal cells that then generate progeny that have luminal features [103] . Alternatively, it may be argued that a malignant phenotype can originate in vivo directly in luminal cells but the conditions used to date simply fail to support this process experimentally. 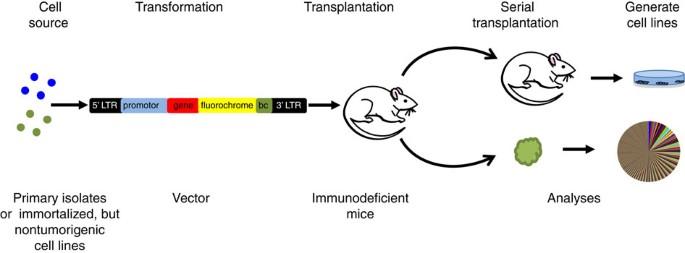Figure 2:De novogeneration of tumours from ‘normal’ human cells. Most examples of successful transformation of primary sources of normal human cells (or non-tumorigenic human cell lines) have used retro- or lenti-viruses encoding one or more oncogenes and a fluorochrome (for example, GFP) to enable malignant cells to be later isolated and characterized. The transduced cells are then transplanted into a receptive site in immunodeficient mice. When a tumour forms, the cells can then be removed for morphological, immunohistochemical, flow cytomteric and/or various molecular and clonal analyses. When this method is efficient, polyclonal tumours may be generated (as illustrated by the pie chart). Retrieved viable cells can also be further transplanted or may be used to generate cell lines. Figure 2: De novo generation of tumours from ‘normal’ human cells. Most examples of successful transformation of primary sources of normal human cells (or non-tumorigenic human cell lines) have used retro- or lenti-viruses encoding one or more oncogenes and a fluorochrome (for example, GFP) to enable malignant cells to be later isolated and characterized. The transduced cells are then transplanted into a receptive site in immunodeficient mice. When a tumour forms, the cells can then be removed for morphological, immunohistochemical, flow cytomteric and/or various molecular and clonal analyses. When this method is efficient, polyclonal tumours may be generated (as illustrated by the pie chart). Retrieved viable cells can also be further transplanted or may be used to generate cell lines. Full size image Table 1 Examples of de novo tumour models from primary human cell sources. Full size table De novo models of tumorigenesis starting from primary human cells have also now been reported for colon and mammary cells. For example, a recent study demonstrated the formation of tumours in immunodeficient mice transplanted with organoids expanded in vitro from colon cells in which CRISPR/Cas9 was used to generate suppressive mutations in APC , SMAD4 and TP53 and activating mutations in KRAS and PIK3CA [104] . De novo genesis of human breast tumours has also now been achieved in immunodeficient mice transplanted with primary isolates of normal cells transduced with p53(R175H) , CCND1 , PIK3CA and KRAS(G12V) [105] , SV40 plus KRAS(G12V) [106] , and more recently with just KRAS(G12D) alone [107] . However, in contrast to the results described for the prostate model, immunohistological analyses of these human breast tumours has indicated the presence of a mixture of phenotypes, possibly related to the polyclonal composition of the tumours generated [107] . The robustness of these models and speed of the tumorigenic process in at least some cases should make them useful for future elucidation of the minimal cellular and extrinsic factors required for their genesis. Examples of de novo leukaemogenesis using primitive (CD34 + ) subsets of hematopoietic cells isolated from human cord blood is also accruing. In this case, examples of genes whose vector-mediated forced overexpression in normal cells have produced overt leukaemic populations in immunodeficient mice include cDNAs for MLL-AF9 (refs 108 , 109 ), MLL-AF4 (ref. 110 ), MN1 plus NUP98HOXD13 (ref. 111 ), BCR-ABL plus a dominant-negative form of IKAROS [112] , and MYC plus BCL [113] . The mixed lineage leukaemia ( MLL ) gene is rearranged and fuses with multiple partner genes in both spontaneously arising human AML and acute lymphoid leukemia (ALL), but the MLL-AF9 fusion oncogene is associated almost exclusively with AML in humans [108] . Interestingly, overexpression of MLL-AF9 in normal cord blood cells produced ALL in transplanted Non-obese diabetic-Scid (NOD-SCID) hosts, but AML in NOD-SCID mice that had been engineered to express three human growth factors. This result illustrates the ability of external factors to dictate the phenotype of the malignant cells produced and further underscores the fallacy in assuming the predominant cell type necessarily reflects the cell of origin or the specific oncogene driving the tumorigenic state. The MN1-NUP98HOXD13 model also serves to illustrate the difference between effects obtained in analogous mouse and human target cells. In mouse cells, MN1 alone was sufficient to induce a myeloid leukaemia, whereas in human cord blood cells it induced only a transient myeloproliferation. Only when an activated HOX gene (that is, NUP98HOXD13 ), was also introduced was a serially transplantable AML obtained in the human cells. These studies demonstrate some of the unique aspects of tumorigenesis in primary human cells that are not well predicted by mouse models. They also provide examples of experimentally generated de novo human tumours whose characteristics are heavily influenced by factors beyond the cell of origin, or the genetic alterations used. Functional diversity of human tumour subclones Most studies attempting to analyse the subclonal diversity of malignant human populations that arise in patients have relied on retrospective inferences derived from analyses of the genomic or phenotypic characterization of primary samples and/or changes incurred in serial transplants of these cells in immunodeficient mouse hosts [23] , [114] , [115] , [116] , [117] , [118] . However, these approaches generally do not allow the frequency of clonogenic cells to be quantified, nor the definition of their genomic or phenotypic properties. These are important parameters because the genomic instability of many established neoplastic human populations can produce genetic alterations that are irrelevant to the continued growth of the tumour. Examples of such mutations have been well documented in genetic analyses of the leukemic cells from patients with chronic phase CML [119] . Limiting dilution analysis (LDA) and vector-based tracking of clonogenic cells offer powerful approaches to quantify malignant cells with proliferative potential in vivo . The LDA approach has been extensively applied to a number of primary human tumour types that can engraft immunodeficient mice. These include malignant populations that arise in the human brain [47] , [120] , colon [48] , [121] , prostate [122] , breast [46] , ovary [123] , skin/melanoma [54] , [124] and the hematopoietic system [45] , [125] , [126] , [127] , [128] . Coupling these approaches to prospectively isolated phenotypes of cells within the transplanted populations has been the basis of identifying the subset(s) of cells actually possessing the tumorigenic activity detected in the recipients. However, to exploit this approach to characterize the clonal growth properties of single tumorigenic cells, the transplants must be initiated with cell numbers that produce tumours at a frequency of less than one in three mice. The large numbers of mice required to obtain clonal data can thus become rapidly prohibitively expensive, if not impractical, particularly when clonal outputs may vary quantitatively as well as phenotypically and dynamically within and between different primary tumours being assessed. The use of massively parallel DNA sequencing has improved the sensitivity and efficiency of vector insert analysis to identify clones based on their semi-random integration sites [129] , thus circumventing many of the limitations of LDA approaches. Nevertheless, ∼ 50% of insertion sites are still elusive to detection using the latest versions of this methodology [129] . A more recent alternative has been the creation and use of libraries of DNA barcoded lentiviral vectors [130] . When such libraries are used at a concentration that results in the transduction of less than one in three cells in the target population being interrogated, and the diversity of the library is greater than the number of cells being investigated, the likelihood that each of the initially marked cells contains a unique barcode is high. The frequency of each barcode in the DNA extracted from populations derived from barcoded cells can then be used to infer the number of cells present in different clones. For both vector strategies, phenotypic purification of the cells to be analysed before extracting the DNA for insert site or barcode analysis allows the phenotypic composition of each clone to also be characterized [109] , [131] , [132] , [133] , [134] , [135] , [136] , [137] . Application of these protocols has revealed complex clonal dynamics in human tumours derived from serially passaged cells [131] . Interestingly, this exercise has documented highly diverse growth behaviours of single cells from cell lines when large numbers of these are transplanted, even though single-cell transplant experiments indicate more than one third can generate a tumour. Thus, to relate the growth activity of the clones with their genotype, it is necessary to isolate and sequence the individual clones generated, as has been done in human glioblastoma [138] . Technological advances are well known to be the drivers of new information. Nowhere is this more relevant than to current issues of interest in the general arena of biomedicine. In the field of human cell oncogenesis, three technologies are of particular relevance: organoid cultures, reprogramming and CRISPR/Cas9. Organoid culture systems are allowing more faithful tissue development to be generated from primitive normal cells and are showing promise for supporting the expansion in vitro of cells derived directly from human tumours [139] , [140] , [141] . Reprogramming allows permanent clonal lines of induced pluripotent stem cells (iPSCs) to be generated from individual malignant cells. CRISPR/Cas9 enables the use of precise gene editing to create new models of human tumours and to test the role of specific genetic alterations in establishing or maintaining the transformed status of patient-derived malignant cells. Organoids This term refers to 3D structures generated in suspension cultures under conditions where 2D growth of attached cells is blocked or prevented (either by suspending the cells in a semi-solid medium-like matrigel or the use of a culture container that prevents cell attachment). The generation of 3D organoids to engineer tissues that are histologically and functionally more similar to their in vivo counterparts will facilitate the modelling of human disorders, performing drug screens, and the creation in vitro of replacement tissues and/or organs. Methods combining directed differentiation of cells in culture systems that promote organoid formation are being developed for many complex tissues such as the liver, kidney, intestine, eye, and brain, to name a few [142] . The advantages of human organoid cultures include better control of the cellular milieu than is associated with tumorigenesis in vivo , better spatial organization of cell types than is achieved in 2D in vitro systems and improved mimicry of in vivo cell behaviour, potential for larger scale testing of variables and drug effects, and reduced ethical concerns and costs associated with animal xenograft experiments. Induced pluripotent stem cells iPSC technology offers a novel method of capturing the genomic state of single cells from almost any source, including transformed cells. However, this comes at the cost of losing the malignant phenotype of the original cells from which each iPSC clone is derived. Nevertheless, from the limited experience where it has been applied to the study of cancer to date, it appears that at least some properties of the malignant cells of origin may be reactivated by stimulating the iPSCs to differentiate back into the lineage or tissue from which the malignant cells arose and may then also be used for drug screening [143] , [144] . iPSCs have been derived from human chronic phase CML cells with documented retention and expression of the signature BCR-ABL1 fusion gene [145] , [146] , [147] . Additional examples of human hematopoietic cells from which iPSCs (or iPSC-like cells) have been obtained include cells from patients with MDS [148] , polycythemia vera [149] and juvenile myelomonocytic leukemia [150] , as well as originally normal human hematopoietic cells forced to overexpress MLL [151] . iPSCs have also been generated from human pancreatic ductal adenocarcinomas [152] , Multiple endocrine neoplasia type 2A (MEN2A) [153] , bladder cancer cell lines [154] and cells from an individual with Li Fraumeni syndrome, a congenital cancer predisposition genotype in which one allele of the p53 gene is mutated [155] . In this case, the iPSCs were used to study the epigenetic states of tumour formation [156] and the bidirectional reversibility of epigenetic processes associated with iPSC reprogramming [157] . CRISPR/Cas9 The CRISPR/Cas9 technology originates from type II CRISPR-Cas systems that evolved to provide bacteria with a form of adaptive immunity to viruses and plasmids. The CRISPR-associated Cas9 protein is an endonuclease that introduces a site-specific double-strand break (DSB) into DNA. The ability of CRISPR/Cas9 to introduce DSBs at defined positions using a guide RNA can also be used to generate human cell lines and primary cells bearing chromosomal translocations resembling those described in human cancers ( Fig. 3 ). Examples to date include lung cancer [158] , AML [159] and Ewing’s sarcoma [160] . An improved method to generate models of liver cancer or myeloid malignancy in mice using CRISPR/Cas9 was also recently reported [161] , [162] . Combining CRISPR/Cas9 with barcoding has been used to track the clonal dynamics of lung cancer cells during their acquired resistance to EGFR inhibitors and subsequent response to combined drug therapies [163] , [164] . Combining the generation of iPSCs with CRISPR/Cas9 holds the future possibility of both creating new models of human cancer and of testing the ultimate therapeutic potential of gene-targeting approaches. 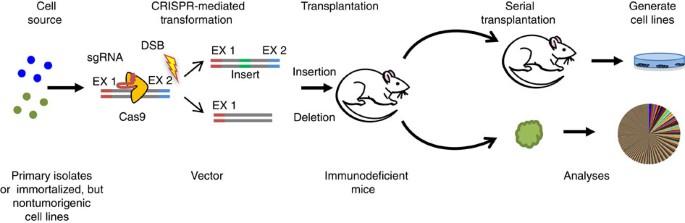Figure 3: Use of>CRISPR/Cas9gene editing to examine the tumorigenic consequences of modifying specific genes in human cells. In this methodology, the test cells are exposed to CRISPR/Cas9 reagents and then transplanted into immunodeficient mice as inFig. 2. Figure 3: Use of> CRISPR/Cas9 gene editing to examine the tumorigenic consequences of modifying specific genes in human cells. In this methodology, the test cells are exposed to CRISPR/Cas9 reagents and then transplanted into immunodeficient mice as in Fig. 2 . Full size image Recreating the process of human tumorigenesis in naive human cells has been a challenging frontier not anticipated by the historically contrasting ease of achieving this outcome in mouse cells. However, several major developments are now changing this picture. One has been the generation of long-lived mice in which multiple components of the innate and acquired immune system have been suppressed. This advance now allows transformed human cells to grow and evolve into fully malignant populations in an in vivo setting. Together with improvements in lentiviral design and production, and methods to isolate and purify normal viable human cells, these advances are now enabling a growing number of de novo models of human tumorigenesis to be developed. The use of DNA barcoding of the initial cells is now also providing a tractable method to analyse the clonal composition and dynamics of the malignant cells generated and should provide a powerful approach to examine therapeutic effects in the future. These approaches coupled with emerging methods to modify and regulate cell behaviour even more precisely herald a new era of improved understanding of the complex processes of human tumorigenesis. How to cite this article: Balani, S. et al . Modeling the process of human tumorigenesis. Nat. Commun. 8 , 15422 doi: 10.1038/ncomms15422 (2017). Publisher’s note: Springer Nature remains neutral with regard to jurisdictional claims in published maps and institutional affiliations.